Murine interfollicular epidermal differentiation is gradualistic with GRHL3 controlling progression from stem to transition cell states 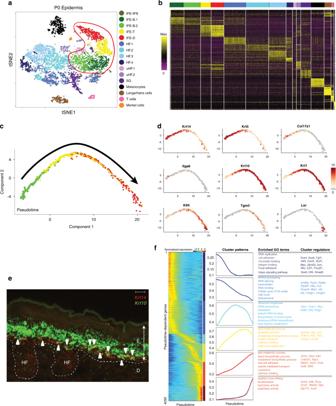Fig. 1: IFE differentiation is gradualistic and features numerous transition cells. atSNE plot showing all 16 epidermal subpopulations of the WT P0 mouse back epidermis; IFE cells are in the red-outlined box. HF hair follicle, uHF upper hair follicle, SG sebaceous gland.bHeatmap showing the expression of top 20 marker genes for all 16 epidermal subpopulations. Gene lists in Supplementary Data1.cPseudotime analysis of the IFE with cluster identity fromaprojected on the trajectory. The trajectory goes from basal to transition to differentiated cells without major branches (arrow), consistent with unidirectional IFE differentiation.dExpression of canonical markers for distinct stages of epidermal differentiation.eRNA-FISH forKrt10andKrt14in WT P0 mouse epidermis. White arrowheads point to yellowKrt10/Krt14double-positive cells. E epidermis, D dermis, HF hair follicle. Scale bar = 10 µm, representative image forN= 5.fExpression heatmap and expression pattern of 4,292 pseudotime-dependent genes that cluster into six gene modules. Also shown are the gene ontology and example transcription factors for each gene module. Gene lists in Supplementary Data1. The interfollicular epidermis (IFE) forms a water-tight barrier that is often disrupted in inflammatory skin diseases. During homeostasis, the IFE is replenished by stem cells in the basal layer that differentiate as they migrate toward the skin surface. Conventionally, IFE differentiation is thought to be stepwise as reflected in sharp boundaries between its basal, spinous, granular and cornified layers. The transcription factor GRHL3 regulates IFE differentiation by transcriptionally activating terminal differentiation genes. Here we use single cell RNA-seq to show that murine IFE differentiation is best described as a single step gradualistic process with a large number of transition cells between the basal and spinous layer. RNA-velocity analysis identifies a commitment point that separates the plastic basal and transition cell state from unidirectionally differentiating cells. We also show that in addition to promoting IFE terminal differentiation, GRHL3 is essential for suppressing epidermal stem cell expansion and the emergence of an abnormal stem cell state by suppressing Wnt signaling in stem cells. During development, the epidermis emerges from the surface ectoderm as a single layer of unspecified progenitor cells, which later form the stratified interfollicular epidermis (IFE), the hair follicles, the sebaceous glands, and the tactile sensing Merkel cells. Meanwhile, mesoderm-derived immune cells and neural crest-derived melanocytes take up residence in the epidermis. Although IFE heterogeneity and differentiation have been previously studied with single cell RNA-sequencing (scRNA-seq) in adult mouse and human skin [1] , [2] , [3] , [4] , [5] , late development of the embryonic IFE has not been studied with scRNA-seq, and key gene regulators of IFE differentiation have not been systematically identified with this method. Conventionally, IFE differentiation is thought to be stepwise as reflected by the IFE’s four distinct layers separated by clear boundaries. Cells of the basal layer, which rest on the basal lamina, are mitotically active stem cells marked by the expression of keratin (K) 5 and K14. As the cells move to the spinous layer, they exit the cell cycle; K5 and K14 expression is replaced by K1 and K10 expression. And as the cells advance to the granular layer, they turn on the expression of barrier-forming genes, including loricrin and filaggrin [6] . Eventually, the terminally differentiated cells cease transcriptional activities and die, flattening and de-nucleating to form the watertight cornified layer that is eventually shed from the skin surface. The layered structure of the epidermis suggests that molecular switches could sharply alter the expression of many genes at the boundaries of distinct cell layers. This prediction, however, has not been studied at a genome-wide scale in the postnatal day (P) 0 mouse epidermis, which—similar to the human epidermis, but in contrast to the adult mouse epidermis—contains clearly demarcated epidermal layers. Layer-restricted expression of transcription factors is thought to contribute to the IFE differentiation program. One such transcription factor, GRHL3, is expressed throughout the developing epidermis during embryogenesis, but becomes restricted to the differentiated layers at P0. Grhl3 -deleted mice have a defective epidermal barrier with decreased expression of cell–cell adhesion molecules, lipid producing enzymes, and proteins required for cornified envelope formation and crosslinking [7] , [8] . At P0, the Grhl3 −/− IFE contains a disorganized basal layer, thickened spinous and granular layers, and a compacted cornified layer. Based on these findings, it has been assumed that the main embryonic role of GRHL3 is to activate genes required for full differentiation of cells of the granular layer. But the nature of the IFE hyperplasia in the P0 Grhl3 −/− mice remains enigmatic. To better understand epidermal differentiation, we investigate single cell transcriptomes from mouse skin during embryogenesis and up to P0 in wild type (WT) and Grhl3 − / − mice. Our findings challenge the classical notion of a stepwise IFE differentiation, which assumes that cells within a layer are relatively uniform but undergo dramatic changes as they move to the layer above. Rather, we find a high proportion of transition cells with a character intermediate between the basal and the first spinous layer, as well as other features suggesting that IFE differentiation is best viewed as a single-step gradualistic process. RNA velocity analysis, though, indicates that prior to the transition-differentiation cell state boundary, cell states are plastic, whereas after this commitment point, cells states proceed strongly in a unidirectional manner toward terminal differentiation. As expected, we find defective activation of terminal differentiation in Grhl3 − / − mice. But unexpectedly, we find accumulation of epidermal stem cell populations and the emergence of proliferative cell states unique to the mutated epidermis. We show that the aberrantly expanded stem cell compartment exhibits increased Wnt signaling while the suprabasal cells exhibit reduced Wnt antagonist expression, with GRHL3 directly binding to key Wnt signaling components. Thus, GRHL3 plays an important role in tempering Wnt signaling and expansion of IFE stem cells during epidermal differentiation. scRNA-seq reveals newborn mouse epidermal cell heterogeneity We started our study into IFE differentiation at a single cell level by focusing on the WT P0 IFE. At this stage, the IFE has reached its maximum thickness with morphologically well-defined layers: basal, spinous, granular, and cornified. We generated single cell transcriptomes from the back epidermis, capturing 5494 cells with 38,879 mean number of reads per cell and 2388 mean number of genes per cell. Clustering identified 16 subpopulations of epidermal cells (Fig. 1a ). Each cluster was annotated by marker genes that are known to be uniquely expressed in each cell type or cell state (Fig. 1b ; Supplementary Fig. 1A–C ). We identified all previously defined epidermal subpopulations of the adult epidermis [2] : IFE, hair follicles, sebaceous gland cells, Langerhans cells, T cells, melanocytes, and Merkel cells (Fig. 1a, b ). Four adjacent clusters of 1779 IFE cells were identified: two basal clusters (IFE.B1 and IFE.B2; 1002 cells), a basal-suprabasal transition cluster (IFE.T; 350 cells), and a differentiated cluster (IFE.D; 427 cells). The population of transition cells (IFE.T) is 20% of the all IFE cells, which is a surprisingly large fraction. The Gene Ontology (GO) category enrichment [9] , [10] of the marker genes of the IFE subpopulations indeed reflects the biological functions of each population (Supplementary Fig. 1D–F ). Fig. 1: IFE differentiation is gradualistic and features numerous transition cells. a tSNE plot showing all 16 epidermal subpopulations of the WT P0 mouse back epidermis; IFE cells are in the red-outlined box. HF hair follicle, uHF upper hair follicle, SG sebaceous gland. b Heatmap showing the expression of top 20 marker genes for all 16 epidermal subpopulations. Gene lists in Supplementary Data 1 . c Pseudotime analysis of the IFE with cluster identity from a projected on the trajectory. The trajectory goes from basal to transition to differentiated cells without major branches (arrow), consistent with unidirectional IFE differentiation. d Expression of canonical markers for distinct stages of epidermal differentiation. e RNA-FISH for Krt10 and Krt14 in WT P0 mouse epidermis. White arrowheads point to yellow Krt10 / Krt14 double-positive cells. E epidermis, D dermis, HF hair follicle. Scale bar = 10 µm, representative image for N = 5. f Expression heatmap and expression pattern of 4,292 pseudotime-dependent genes that cluster into six gene modules. Also shown are the gene ontology and example transcription factors for each gene module. Gene lists in Supplementary Data 1 . Full size image The IFE consists of numerous basal-spinous transition cells To gain greater insights into the progression of IFE differentiation at P0, we next applied pseudo-temporal analysis. We used Monocle [11] , an algorithm that uses changes in gene expression between cells to learn in an unbiased manner the position of each cell in a biological trajectory. Monocle introduces the concept of pseudotime as an abstract measure of how far a cell has progressed in a process—here in the differentiation of an IFE stem cell in the basal layer to a terminally differentiated keratinocyte at the top of the epidermis. Monocle ordered the IFE cells along a linear trajectory without introducing significant bifurcations (Fig. 1c ). This differentiation trajectory corresponds well with our cluster annotation from Fig. 1a in that the cells progress from IFE.B through IFE.T to IFE.D. To validate the pseudotime ordering, we assessed the expression of canonical markers in the trajectory (Fig. 1d ), finding that K14/K5/Col17a1/Itga6 mark cells in the early trajectory, K10/K1/Klf4/Tgm3 in the middle-to-end trajectory, and Lor in the end of the trajectory. These results suggest that Monocle ordered the IFE keratinocytes in a biologically meaningful manner from the most undifferentiated to the most differentiated cells. We noted high number of transition cells with falling K5/K14 expression and rising K1/K10 expression—characteristics that are intermediary between the basal and spinous layers. This finding is unexpected because of the apparent sharp boundary between the basal and spinous layer [12] . To validate the existence of the transition cells, we performed RNA FISH with Krt14 and Krt10 probes. Consistent with the scRNA-seq data, we observed a substantial number of double positive transition cells both in the basal and in the first spinous layer (Fig. 1e ). These results indicate that (1) epidermal differentiation has already begun in the basal layer [13] , (2) some spinous cells still retain basal characteristics, and (3) a relatively large population of transition cells exists at the basal-spinous boundary. The IFE differentiates gradually in a single-step To better understand differentiation at a molecular level, we identified 4299 genes that are dynamically expressed over the pseudotime trajectory. 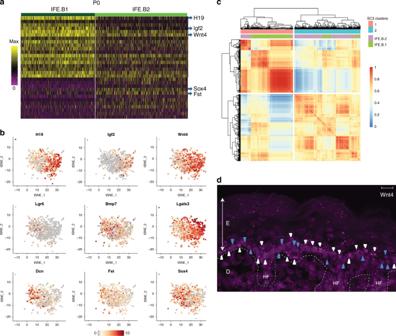Fig. 2: The P0 IFE basal cell layer contains two distinct cell populations. aExpression heatmap of unique gene signatures for each of the two basal IFE clusters. Blue arrows highlight select differentially expressed genes between the two basal clusters. Gene lists in Supplementary Data1.bExpression level of select genes, which are enriched in either IFE.B1 or IFE.B2, projected onto tSNE for the two basal clusters.cHeatmap showing the correlation between cells for SC3 clustering (1, 2; red, blue) and Seurat clustering (IFE.B1, IFE.B2; purple, green).dRNA-FISH forWnt4in the P0 IFE. White arrowheads,Wnt4-high cells; blue arrowheads,Wnt4-low cells; white broken line, basal lamina; E epidermis, D dermis, HF hair follicle. Scale bar = 10 µm, representative image forN= 5. K-medoid clustering grouped these genes into six gene modules with distinct expression patterns and biological functions (Fig. 1f ) [9] , [10] , [14] . Module 1, high early and falls sharply, is enriched in genes associated with cell proliferation. Module 2, also high early but falls more slowly, is enriched in genes involved in transcription and mRNA processing. Module 3, peaks in the middle of the trajectory, is enriched in genes for ribosome biogenesis and protein translation. Module 4, peaks towards the end, is enriched in lipid biosynthesis genes. Module 5, also peaks toward the end but with a slower rise, is also enriched in lipid synthesis pathways and in cell adhesion genes. Module 6, a sharp peak at the end, is enriched in crosslinking and barrier genes. Each module contains transcription factors with known functions in IFE differentiation that match the overall gene functional category of that cluster. At early differentiation stages, transcription factors associated with the cell cycle and DNA repair are highly expressed, including Trp53, Smad4, Hmgb1 , and Hmgb2 . As differentiation commences, Mafb and Myc become highly expressed whereas late differentiation transcription factors such as Klf4 and Grhl3 become highly expressed at late and terminal differentiation stages. In addition, we have identified many candidate transcription factors with heretofore unknown roles in the IFE (Fig. 1f ). Although these findings correspond well with known features of IFE differentiation, they also point to an unusual relationship between cell proliferation and protein synthesis which are normally tightly coupled; in the IFE, peak gene expression for protein synthesis appears after peak expression of cell cycle genes. Furthermore, these data indicate that the majority of IFE differentiation genes exhibit expression that is not layer-specific with at least four out of six gene modules straddling different layers. This result and the observed high number of transition cells challenge the traditional model of stepwise IFE differentiation, suggesting that at a transcript level, IFE differentiation is continuous and gradualistic. The IFE basal layer contains two distinct cell populations Next we sought to better decipher P0 basal IFE stem cell heterogeneity by examining the unique molecular signatures expressed in the two basal subpopulations (Figs. 1 a and 2a ). IFE.B1 cells (446 cells) express H19 , Igf2 , and Wnt 4 at a higher level than IFE.B2 cells, whereas IFE.B2 cells (556 cells) exclusively express Sox4 and Fst , as well as other markers, including Dcn (Fig. 2a, b ). We performed principle component analysis (PCA) on these two populations and found the above markers to be among the genes that explain most of the variances in the first PC (Supplementary Fig. 2A ); in contrast, cell cycle genes do not contribute to variances in the first few PCs. To confirm that active cell cycling does not play a major role in defining the two basal clusters, we also regressed out the cell cycle genes and reclustered the basal IFE cells, which did not alter the results (Supplementary Fig. 2B–D ). Therefore, we ruled out the possibility that these clusters are due to differences in cell cycle stages among the cells. Furthermore, IFE.B1 and B2 are not distinct stages of differentiation on the pseudotime trajectory (Supplementary Fig. 2E ). In addition, we used an independent clustering method, SC3 [15] , to recluster all basal IFE cells; SC3 clustering results were very similar to Seurat’s, confirming the robustness of this finding (Fig. 2c ). Fig. 2: The P0 IFE basal cell layer contains two distinct cell populations. a Expression heatmap of unique gene signatures for each of the two basal IFE clusters. Blue arrows highlight select differentially expressed genes between the two basal clusters. Gene lists in Supplementary Data 1 . b Expression level of select genes, which are enriched in either IFE.B1 or IFE.B2, projected onto tSNE for the two basal clusters. c Heatmap showing the correlation between cells for SC3 clustering (1, 2; red, blue) and Seurat clustering (IFE.B1, IFE.B2; purple, green). d RNA-FISH for Wnt4 in the P0 IFE. White arrowheads, Wnt4- high cells; blue arrowheads, Wnt4 -low cells; white broken line, basal lamina; E epidermis, D dermis, HF hair follicle. Scale bar = 10 µm, representative image for N = 5. Full size image Our data, then, highlight IFE basal cell heterogeneity, suggesting there are two basal stem cell populations in the P0 IFE. To validate our findings, we carried out RNA-FISH studies with H19 and Wnt 4 probes. We found that Wnt 4-high and Wnt 4-low cells are distributed heterogeneously within the IFE basal layer (Fig. 2d ) and that high H19 expression tends to co-localize with the Wnt 4-high cells (Supplementary Fig. 2F ). These findings indicate that the IFE.B1 and IFE.B2 cells intermingle in the basal layer and are not spatially distinct groups of cells. Our findings are in agreement with previous studies showing that Wnt-secreting stem cells play a central role in IFE self-renewal during homeostasis [16] , [17] , [18] . The IFE differentiation program is established at E14.5 To investigate when the above-described characteristics of the IFE appear and how the differentiation program may change during development, we generated single cell suspensions from littermate WT and Grhl3 −/− mouse dorsal whole skin (E14.5, E16.5) and epidermis (E18.5/P0). We then performed scRNA-seq on two biological replicates from each time point for each genotype (Supplementary Figs. 3A–F , 4A–F , and 5A, B ). In our computational analysis, we focused first on normal IFE development, selecting IFE cells from all three time points (Fig. 4a , Supplementary Fig. 3A) and clustering them jointly into six cell states (Fig. 3a–c ) based on canonical markers of IFE differentiation (Fig. 3c ). We observed basal, transition, spinous, and terminally differentiated IFE clusters at each of the three developmental time points, indicating that the full IFE differentiation program is functional as early as E14.5 (Fig. 3a ). Fig. 3: The IFE Differentiation program is already established at E14.5. a UMAP showing distribution of cell states as defined in the P0 IFE (Fig. 1 ) in the developing IFE (E14.5, E16.5, and P0). We observe two transition populations, IFEE.T1 and IFE.T2, at E14.5 and E16.5. IFE.T2 cells are proliferating transition cells. b Pie charts showing the proportion of major cell states at each developmental time point. IFE.B and IFE.TD decrease and increase, respectively, across development. c The expression of the indicated differentiation and proliferation markers projected onto the combined UMAP for all three developmental time points in a . d PHATE maps of cell populations defined in a , showing pseudotime progression at each developmental stage. The gray circle emphasizes the extension of terminal differentiation at P0. e Expression of the indicated differentiation and proliferation markers onto the combined PHATE maps from d . f Left panel, expression heatmap and expression pattern of 2801 pseudotime-dependent genes from the combined PHATE maps from d ; these cluster into six gene modules. Right panel, expression heatmap of 149 pseudotime-dependent transcription factor (TF) genes from the combined PHATE maps from c . Representative TFs from each gene modules are color-coded and indicated on the left. Gene lists in Supplementary Data 1 . g Gene ontology categories of genes differentially expressed at each developmental stage in all IFE cells. Gene lists in Supplementary Data 1 . h Gene ontology categories of genes differentially expressed at E16.5 and P0 in IFE.B1 and IFE.B2 cells. Gene lists in Supplementary Data 1 . i Gene ontology categories of genes differentially expressed at E16.5 and P0 in IFE.D and IFE.TD cells. Gene lists in Supplementary Data 1 . Full size image Even though we observed the full range of IFE differentiation states across the developmental time points, there are changes in the proportion of cell states when comparing the E14.5 with the P0 IFEs (Fig. 3b ). The proportion of basal cells decreases as the skin develops (IFE-B; 52% at E14.5, 58% at E16.5, 37% at P0). In contrast, the proportions of transition cells (IFE-T; 19% at E14.5, 19% at E16.5, 23% at P0), differentiated cells (IFE-D; 22% at E14.5, 15% at E16.5, 27% at P0), and terminally differentiated cells (IFE-TD; 7% at E14.5, 8% at E16.5, 13% at P0) all increase. The E14.5 IFE.T cells, however, are different from IFE.T cells of the P0 IFE in that the E14.5 IFE.T cells are highly proliferative (Fig. 3c and Supplementary Fig. 3G, H ), consistent with known features of the intermediate layer at this developmental stage. We observed this feature to a lesser extent for the E16.5 IFE.T cells (Fig. 3c and Supplementary Fig. 4G, H ). The pseudotemporal ordering of E14.5 and E16.5 IFE cells separately shows linear trajectories with a single branch consisting mostly of proliferating IFE.T cells (Supplementary Figs. 3G and 4G ). This finding corroborates the idea that IFE cells goes through a state of rapid proliferation before differentiating at E14.5, a feature that decreases at E16.5, and is abolished at P0. scEpath pseudotemporal trajectory analysis [14] on the integrated data from all three developmental time points revealed a linear differentiation trajectory with a small outlying cluster mainly composed of proliferative IFE.T cells from E14.5 and E16.5 (Fig. 3d, e ). Consistent with our clustering results, the distal end of the trajectory containing IFE.TD cells extends further in the P0 than the E14.5 and the E16.5 IFEs (Fig. 3d ). Across this integrated trajectory, 2801 genes show pseudotime-dependent change in expression; these can be grouped into six gene modules, which contain 149 transcription factors (Fig. 3f ). To investigate how gene expression programs change during IFE development, we compared the differentially expressed genes in IFE cells across the three time points. We found that in IFE cells collectively, E14.5 and E16.5 cells display higher expression of genes for growth, nucleic acid metabolism, and RNA regulation, whereas P0 cells display higher expression of genes for cell–cell adhesion and barrier formation (Fig. 3g ). In IFE.B cells selectively, there is enrichment for cell cycle and cell migration at E16.5, whereas there is greater enrichment for nuclear division and cell growth at P0 (Fig. 3h ). In IFE.D and IFE.TD cells, there is enrichment for myeloid cell differentiation, cytokine secretion and ERK signaling at E16.5, whereas there is enrichment for lipid metabolism and morphogenesis at P0 (Fig. 3i ). Taken together, these data indicate that the full range of the IFE differentiation program is already established as early as E14.5, and that epidermal development from this time point is characterized by a subtle shift toward differentiated cell states and away from growth and proliferation. GRHL3 is required for tempering IFE stem cell number Previous work on GRHL3 suggested that all layers of the IFE do develop in Grhl3 − / − embryos, although at P0 the basal layer is disorganized and the spinous and granular layers appear thicker than normal [7] , [8] . Bulk gene expression measurement and other studies suggested that GRHL3 transcriptionally activates the terminal differentiation gene expression program in the granular layer [7] , [8] . The differentiation-specific function of GRHL3 is also consistent with the restricted expression of GRHL3 in the most differentiated layers of the IFE at P0. How GRHL3 affects IFE cell states has not been investigated. Hence, we tested how GRHL3 affects P0 IFE differentiation as detected by scRNA-seq. We performed scRNA-seq on single cell suspensions from the back-skin epidermis of two WT and two Grhl3 −/− littermates at P0, capturing a total of 29,796 cells after quality control (WT1 = 6766, WT2 = 6590, Grhl3 − / − 1 = 9157, Grhl3 − / − 2 = 7283) (Supplementary Fig. 5A, B ). As expected, we recaptured the IFE cell heterogeneity depicted in Fig. 1 (Fig. 4a, b ), including the basal keratinocyte heterogeneity, thus validating these earlier findings (Figs. 1 and 2 ). But here, we identified a third, actively proliferating basal population (IFE.B3) (Fig. 4a and Supplementary Fig. 5c ); this cluster most likely emerged due to increased total number of cells captured across the four samples compared to the experiment in Figs. 1 and 2 . We also believe that the higher number of cells included in this experiment allowed the terminally differentiated (IFE.TD) IFE cells to form a distinct cluster. Fig. 4: GRHL3 is required for suppressing aberrant basal IFE stem cells. a tSNE plot showing WT and Grhl3 −/− P0 IFE cells colored by clusters (left) and genotype (right). b Bar plot showing the fraction of each IFE cell type in each sample. There is expansion of basal cells and reduction of differentiated/terminally differentiated cells in Grhl3 − / − IFE. c Gene expression levels of markers for the IFE.A1 population. Sprr2a3, Tpm2, Ly6a and Eif3 are shown on a tSNE plot of the P0 IFE cells. d Representative RNA-FISH of Krt14 and Krt10 transcripts in P0 WT and Grhl3 − / − mouse epidermis; white arrows highlight Krt14 / Krt10 double-positive transition cells. Note the higher number of double-positive cells in the Grhl3 − / − epidermis; also some transition cells are found in the spinous layer. N = 5. White broken line, basal lamina; E epidermis, D dermis, HF hair follicle. Scale bar = 10 µm. Full size image We integrated all four samples [19] and found that although the proportion of each of the IFE subpopulations is consistent between the two wild type epidermis, the cell composition of the mutant epidermis is clearly different from the wild type (Fig. 4b ). The terminally differentiated IFE population (IFE.TD) is almost absent in the Grhl3 − / − IFE (Fig. 4a, b ), suggesting that in addition to activating the expression of terminal differentiation genes, GRHL3 promotes the formation of the most differentiated cells of the IFE. Most strikingly, however, the proportion of basal cells (IFE.B1, IFE.B2, and IFE.B3) increased, whereas the proportion of transitioning (IFE.T) and differentiated cells (IFE.D) decreased (Fig. 4b and Supplementary Fig. 5D ) in the Grhl3 − / − IFE. In addition, we detected a substantial number of cells representing IFE states that are nearly exclusive to the Grhl3 − / − epidermis. We termed these two populations aberrant IFE 1 and 2 (IFE.A1, IFE.A2). About 100 IFE.A1 cells were found in each of the two Grhl3 − / − biological replicates, whereas a greater number (135) of IFE.A2 cells were found in Grhl3 −/− 2 than Grhl3 −/− 1 (18) (Fig. 4a, b ). We observed no clear changes in cellular composition between WT and Grhl3 − / − IFE cells at E14.5 and E16.5, suggesting that the cell state differences in the Grhl3 −/− IFE arose between E16.5 and P0 (Supplementary Fig. 5E ). These findings indicate that in addition to promoting terminal differentiation, a major function of GRHL3 is to suppress the abundance of epidermal stem cells and the formation of abnormal IFE cell states at the later stages of IFE development. GRHL3 suppresses aberrantly differentiated IFE progenitors The IFE.A1 cells resemble the normal transitioning cell state (IFE.T) in that they express both basal and suprabasal IFE gene signatures (Supplementary Fig. 6A ). Consistently, we find IFE.A1 cells between the basal and differentiated IFE cells on PCA analysis (Supplementary Fig. 6B ). RNA-FISH staining of the IFE showed an increase in the number of cells in the basal and spinous layers expressing both basal ( Krt14 ) and suprabasal ( Krt10 ) markers in the Grhl3 − / − epidermis compared to WT (Fig. 4d ). Immunofluorescence staining corroborates this at the protein level (Supplementary Fig. 6C ), suggesting that the IFE.A1 cells are located at the basal-spinous boundary. Yet, the IFE.A1 population also expresses genes distinct from wild type IFE.T cells, including Sprr2a3 , Tpm2 , and Ly6a (Fig. 4c , Supplementary Fig. 6D ). Furthermore, cell cycle analysis [19] , [20] on all IFE subpopulations revealed that IFE.A1 cells are more proliferative than the IFE.T cells; in fact, a subset of IFE.A1 cells express proliferation genes to a similar level as the dividing basal cluster IFE.B3 (Supplementary Fig. 6E, F ). These findings indicate that GRHL3 suppresses the formation of aberrantly differentiated epidermal progenitors. Given the unexpected change in basal cell composition and the emergence of aberrant transition-like cells in the Grhl3 − / − IFE, we conclude that GRHL3 is required for maintaining proper IFE cell composition, acting as early as the transition state between basal and spinous cells. GRHL3 loss disrupts differentiation at the IFE.B–IFE.T transition To further define the differentiation stage in which GRHL3 functions during IFE differentiation, we constructed separate pseudotime trajectories for WT and Grhl3 − / − IFE cells. In agreement with our earlier experiment (Fig. 1c ), the two WT IFE samples formed a linear trajectory going from basal to terminally differentiated cells (Fig. 5a, b and Supplementary Fig. 7A ). In the Grhl3 − / − IFE, the aforementioned expansion of proliferating basal cells and the presence of the IFE.A1 subpopulation both contributed to a branching of the linear differentiation trajectory (Fig. 5a ). The branching occurred at the junction between basal cells and IFE.T cells. The tip of the aberrant branch in the Grhl3 − / − IFE is composed of highly proliferating basal IFE cells (IFE.B3) and the IFE.A1 cells. Consistent with the Seurat clustering (Fig. 4a ) and the RNA-FISH experiments (Fig. 4d ), this pseudotime analysis also suggests that the IFE.A1 cell state is most similar to that of IFE.T cells. In contrast, the IFE.A2 cells are more similar to cells at a later differentiated stage, albeit with higher proliferation (Supplementary Fig. 6E, F ). The IFE.A2 cells also express mitochondrial genes and other markers of cellular stress (Supplementary Data 1 ), which may explain the variability in this cell population between the two replicates; we speculate that the IFE.A2 population may be a sensitive marker of the cellular damage associated with hyperproliferation and defective barrier. In sum, besides being a transcriptional activator of late differentiation genes, GRHL3 performs important functions at early stages of IFE differentiation. Fig. 5: RNA velocity reveals a commitment point at the IFE.T/IFE.D transition. a Pseudotime trajectories showing IFE differentiation going from IFE-B to IFE-T to IFE-D to IFE-TD for the two WT (left) and two Grhl3 − / − (right) P0 IFEs. The Grhl3 − / − differentiation trajectory has a branch which is attributed to the IFE-A1 population and expansion of basal, proliferating cells. b Expression of Krt14 , Krt5 , Krt10 , and Krt1 projected on the pseudotime trajectory for the WT (left) and the Grhl3 − / − (right) IFE. c RNA-Velocity analysis of the pseudotime trajectory of IFE cells for WT1, WT2, Grhl3 − / − 1, Grhl3 −/− 2. Direction of the arrows points to the fate the cells are heading toward; length of the arrows reflects how fast the cells are heading toward a particular fate. Note IFE differentiation is marked by a clear commitment point (arrowhead) and is a one-step, continuous process with no intermediary stages in the WT. In contrast, most cells fail to proceed through the commitment point (arrowhead) and transition cells show a propensity to go back to basal fate in the Grhl3 −/− IFE. Full size image RNA-velocity reveals a differentiation commitment point To further understand the differentiation abnormalities in the Grhl3 − / − IFE, we applied RNA-velocity, a method that exploits the relative abundance of nascent (unspliced) and mature (spliced) transcripts to predict the future state of individual cells on a time scale of hours [21] , [22] . This method can infer directionality and dynamics of small groups of cells with respect to each other in the pseudotime differentiation trajectory. In these data, the direction of the arrows point to the fate the cells are heading toward whereas the length of the arrows reflects how fast the cells are heading in that direction. We expected that RNA-velocity would reveal arrows with a uniform direction from IFE.B to IFE.TD in the pseudotime trajectory of the WT IFE. Surprisingly, we found that during WT IFE differentiation, the basal and transition cells exist in a dynamic equilibrium state in which no clear directionality is observed among them (Fig. 5c ). Once the cells reach the IFE.T/IFE.D boundary, the arrows become longer and align in the direction of terminal differentiation in a uniform manner, suggesting that after cells exit the IFE.T state, they commit to differentiate in a uniform manner until they terminally differentiate (Fig. 5c ). These results are not exclusive to this particular dimension reduction method as we found similar results with PCA of all IFE cells, which also happens to delineate IFE’s linear differentiation trajectory from IFE.B to IFE.T to IFE.D (Supplementary Fig. 7B ). In the Grhl3 − / − IFE, much fewer cells pass the IFE.T/IFE.D commitment point where unidirectional IFE differentiation commences. Strikingly, early transition cells display a clear propensity back toward the basal cell fate, again suggesting that GRHL3 plays an important role in promoting the differentiation of IFE.B to IFE.T cells. These findings suggest: (1) Normal IFE differentiation proceeds in a smooth, continuous manner rather than in punctuated stages. (2) There are crucial changes in the regulation of IFE differentiation at the IFE.T/IFE.D boundary, where cells commit to differentiate and at which GRHL3 plays a key role. (3) Early progenitor cells transitioning to differentiation are highly plastic in their progenitor-differentiation fate decisions. (4) There is aberrant signaling in the Grhl3 − / − epidermis that actively drives early transition cells toward the basal fate. GRHL3 represses Wnt signaling in the IFE In the P0 Grhl3 −/− IFE, the basal compartment is expanded (Fig. 4b ) and IFE.T cells exhibit a propensity to go backward toward the basal fate as shown with RNA velocity analysis (Fig. 5c ). These findings suggest that GRHL3 is required for suppressing signaling pathways that actively drive IFE cells toward the basal fate. Previous mouse experiments showed that Wnt-secreting keratinocyte stem cells are distributed in the basal IFE and that autocrine Wnt signaling is required for self-renewal in mouse adult epidermal homeostasis [16] , [18] . Hence, we hypothesized that aberrant Wnt signaling could explain the change in cell composition and disruption of differentiation in the Grhl3 −/− IFE. To determine if Wnt signaling is altered in the Grhl3 −/− IFE, we compared the expression level of Wnt signaling pathway components between P0 WT and Grhl3 −/− IFE populations in our scRNA-seq data. We observed increased expression of genes such as Wnt4 , Lef1 , Ctnnb1 , Gpc3 , and Gsk3b in the Grhl3 −/− basal IFE populations and the IFE.A (Fig. 6a and Supplementary Fig. 8A ). As Grhl3 is expressed at highest levels in the spinous and granular layers in WT mice, we also considered that GRHL3 could suppress Wnt signaling in a paracrine manner by regulating Wnt inhibitory ligand expression. Consistent with this idea, we found that Dkkl1 , encoding a known Wnt pathway antagonist [23] , is expressed at a high level in the spinous and granular layers but not in the basal layer (Fig. 6b ). In the Grhl3 −/− IFE, Dkkl1 expression level is reduced, as are the number of cells expressing Dkkl1 (Fig. 6b and Supplementary Fig. 8C ). To validate these findings, we performed RNA-FISH for the Wnt ligand Wnt4 and the Wnt downstream effector Lef1 in WT and Grhl3 −/− IFE; both Wnt4 and Lef1 are expressed at a higher level in the Grhl3 −/− IFE (Fig. 6c ). Furthermore, whereas Wnt4 and Lef1 expression is restricted to a subset of basal cells in the WT IFE, they are expressed more widely in basal cells and in cells of the spinous layer in the Grhl3 −/− IFE (Fig. 6c ). In RNA-FISH experiments, we also found that Dkkl1 is expressed at a lower level in the suprabasal compartment of the Grhl3 −/− IFE (Fig. 6d ). These RNA-FISH results are consistent with the scRNA-seq results showing an increase in the number of keratinocyte stem cells (IFE.B) in the Grhl3 −/− IFE and the fact that the IFE.A population, which is enriched in the Grhl3 −/− IFE, is a transition population expressing high level of Wnt4 . Fig. 6: GRHL3 represses Wnt pathway gene expression in basal IFE cells. a Violin plot showing the Wnt4 (left) and Lef1 (right) expression for each cell among the basal cell types in the WT (both biological replicates) and the Grhl3 − / − (both biological replicates) IFE. There is higher number of Wnt4 -high and Lef1 -high cells in all basal and aberrant populations in the Grhl3 − / − than in the WT. b Expression of Dkkl1 projected on the pseudotime trajectory for the WT (top) and the Grhl3 − / − (bottom) IFE. Note the decreased number of cells expressing Dkkl1 in the Grhl3 −/− IFE. c Representative RNA-FISH images of Wnt4 (upper panels) and Lef1 (lower panels) in WT and Grhl3 − / − P0 epidermis. There is increased Wnt4 expression and aberrant expression of Wnt4 in cells above the basal layer in Grhl3 − / − IFE as indicated with white arrowheads. There is increased Lef1 expression in the basal layer in the Grhl3 −/− IFE as indicated with white arrowheads. N = 3 WT and Grhl3 −/− littermates. E epidermis, D dermis, HF hair follicle. d Representative RNA-FISH image of Dkkl1 in WT and Grhl3 − / − P0 epidermis. There is decreased Dkkl1 expression in the suprabasal layers in Grhl3 − / − IFE. N = 3 WT and Grhl3 −/− littermates. White broken lines trace the basal lamina. E epidermis, D dermis, HF hair follicle. Scale bars = 10 µm. Full size image Noting a connection between GRHL3 and Wnt signaling, we explored our previously published GRHL3 ChIP-seq data from the E16.5 epidermis [24] . We found that GRHL3 directly binds to the promoters of key Wnt signaling components, including Wnt4 , Lef1 , Ctnnb1 , Gsk3b and Ctnnbip1 (Fig. 7a and Supplementary Fig. 8B ), and near gene bodies of Axin2 , Myc (Supplementary Fig. 8B ). These data are consistent with GRHL3 directly regulating Wnt signaling to maintain proper balance between proliferation and differentiation in the IFE. Next, we set out to determine if suppressing Wnt signaling can decrease the thickness of the hyperthickened IFE in Grhl3 −/− mice at P0. We harvested P0 mouse back skin and used Wnt-C59, a small molecule antagonist of the Wnt pathway, or DMSO to treat samples from the same skin ex vivo for 48 h in media. Wnt-C59 effectively suppressed Wnt signaling in the epidermis (Fig. 7b ). Meanwhile, the Wnt antagonist significantly decreased the thickness of the hyperplastic Grhl3 −/− IFE (Fig. 7c, d ). Taken together, these results reveal a previously unexpected role of GRHL3 in suppressing Wnt signaling, thereby promoting the transition from basal to transition IFE cells. Fig. 7: Wnt inhibition partially rescues epidermal hyperplasia in the Grhl3 − / − IFE. a GRHL3 ChIP-seq signal on the indicated Wnt signaling genes in the E16.5 epidermis. The red bars represent significant peaks. b Representative RNA-FISH images of Wnt4 (pink) and Lef1 (green) in Grhl3 − / − P0 epidermis treated ex vivo with control (DMSO; left panel) or Wnt inhibitor (Wnt-C59; right panel). There is decreased Wnt4 and Lef1 expression in the epidermis treated with the Wnt inhibitor. Arrowheads point to signal. N = 3 biologically independent samples each. White broken line traces basal lamina. E epidermis, D dermis, HF hair follicle. c Representative sections of Grhl3 −/− P0 epidermis treated ex vivo with control (DMSO; left panel) or Wnt inhibitor (Wnt-C59; right panel), representative image for N = 3 each. Krt14 staining, red; Krt10 staining, green; DAPI staining; blue; HF, hair follicle. There is decreased IFE thickening of the Wnt inhibitor treated epidermis. Scale bar = 10 µm. d Summary statistics for IFE thickness, mean and standard error for ex vivo Wnt inhibitor experiments. P -value was calculated with one-tailed student t -test. N = 3 biologically independent samples each. Full size image Here, we report single cell transcriptome profiling study of the developing mouse epidermis at E14.5, E16.5, and P0 in WT and Grhl3 −/− mice. The data includes a total of 85,286 cells, a valuable resource available for analysis beyond the scope of this paper. We identified all known cell types of the epidermis and defined unique gene signatures for each cell type. We have also uncovered numerous hitherto unknown genes important for IFE differentiation and development from E14.5 to P0. Our study, which focused on IFE differentiation and its regulation by GRHL3, has revealed a number of insights: (1) At a transcript level, IFE differentiation is continuous and gradualistic rather than stepwise (Fig. 1 ); (2) There is a large number of basal-spinous transition cells (Fig. 1 ); (3) An important regulatory change occurs at the IFE.T/IFE.D boundary where IFE cells commit from a plastic state to an irreversible fate toward terminal differentiation (Fig. 5c ); (4) There are two main populations of basal stem cells and a third basal cell state linked to cell proliferation (Figs. 1 , 2 , and 4 ); (5) The full IFE differentiation program is already operating as early as E14.5 (Fig. 3 ); (6) In addition to a role in promoting terminal differentiation in the most differentiated cells, GRHL3 is required at an earlier differentiation stage to suppress Wnt signaling and to suppress the expansion of stem cells (Figs. 4 , 6 , 7 ). Clearly, the IFE contains morphologically distinct layers. Yet, our scRNA-seq findings challenge the conventional notion of stepwise IFE differentiation (Supplementary Fig. 8D ). At a transcript level, differentiation occurs in a continuous manner from the most primitive stem cell to the most terminally differentiated IFE cell at the top of the epidermis. The demonstration of a large number of transition cells also supports the gradualistic model for IFE differentiation. Consistent with previous results, our findings suggest that basal stem cells (IFE.B) exist in a reversible equilibrium with a large population of transition cells (IFE.T) and that is not until after passing the transition cell stage that IFE cells fully commit to differentiation. In the future, live imaging likely will be a powerful tool to investigate the gradualistic feature of IFE differentiation with quantitative, temporal resolution. Studies on stem cells in the basal layer of the adult epidermis have suggested cell heterogeneity within this layer, although the nature of this heterogeneity remains controversial. The hierarchical model of stem cell differentiation suggests that the basal layer comprises rare slow-cycling long-term stem cells and their fast-cycling committed progenitors [25] , [26] . Another related model suggests that slow-cycling and fast-cycling stem cells occupy distinct regions of the basal layer and renew within their respective regions [27] , [28] . By contrast, the stochastic model of stem cell differentiation suggests that all basal cells are equivalent in terms of their stemness and that they differentiate in a stochastic manner [16] , [29] , [30] , [31] . We found two populations of stem cells in the P0 IFE with one major difference between these being the higher expression of Wnt4 in IFE.B1. Wnt4 was previously shown to be important for IFE stem cell self-renewal [16] and our RNA-FISH results also support a model in which Wnt4 -high stem cells are distributed randomly throughout the basal IFE. We propose that Wnt4 -high basal IFE cells are workhorses of IFE maintenance as increased Wnt4 due to Grhl3 loss leads to a considerable change in cell composition of the IFE. Previous work on GRHL3 has focused on suprabasal IFE cells where Grhl3 expression is the highest and where it regulates terminal differentiation genes [7] , [8] . scRNA-seq allowed us to quantitatively characterize the cell compositional change in Grhl3 −/− epidermis and uncover another important function of GRHL3, which is to suppress expansion of IFE stem cells and Wnt signaling in the basal layer. RNA velocity analysis suggests that the intermediate cell state (IFE.T) is plastic and can either revert to the basal stem cell (IFE.B) state or progress toward differentiation (IFE.D). Unexpectedly, we find that GRHL3 promotes the progression of the IFE.B state to the IFE.T state, which accounts for the prominent accumulation of epidermal stem cells in the Grhl3 −/− IFE. Based on our findings of increased Wnt signaling activity in the Grhl3 −/− IFE and on previous work showing that Wnt signaling promotes IFE stem cell proliferation and maintenance [16] , [17] , we postulate that an important developmental role of GRHL3 is to temper Wnt signaling in IFE stem cells. As GRHL3 binds to the promoters of several Wnt signaling genes, including Wnt4 and Lef1 , this effect may be from direct transcriptional repression of key Wnt effectors; we have previously shown that GRHL3 binding to promoters is often associated with transcriptional repression [32] . This model is consistent with data from human keratinocytes suggesting that GRHL3 may act early in maintaining proper proliferation/differentiation balance [33] , [34] . But our scRNA-seq data also suggests that paracrine mechanisms could be at play. The secreted Wnt pathway antagonist DKKL1, which is normally expressed in the terminally differentiated cells of the IFE, is decreased in the Grhl3 −/− IFE, thereby potentially decreasing the suppression of Wnt signaling in the basal layer. Mouse work One male and one female for each genotype (WT (C57Bl/6J), Grhl3 −/− mice [7] ) for each time point were used. Timed pregnancies were used to obtain embryos for E14.5, E16.5, and E18.5; the developmental stage of embryos was verified using external features of the embryos [35] . All experiments were performed on WT and Grhl3 −/− littermates from the same pregnancy. Mice were fed food and water ad libitum and maintained on a regular 12 h day/night cycle. All animal experiments were performed in accordance with Institutional Animal Care and Use Committee at University of California, Irvine (Protocol No. AUP-19-012). Tissue isolation All Grhl3 −/− embryos displayed spina bifida. For E18.5/P0 mice, we removed approximately 6 mm radius circular sample of backskin, centered at the midline in one axis and on a line drawn between the forelimbs in the other axis. The same region of skin was microdissected for E14.5 and E16.5 embryos. This anterior location avoids skin near the spina bifida defect. For E14.5 and E16.5, the micro-dissected embryonic back skin was incubated in 2.5 U/ml Dispase (STEMCELL Technologies) in EpiLife medium (Thermo Fisher Scientific) for 2 h at room temperature (RT). The tissue were then washed with media and incubated in Accutase (STEMCELL Technologies) for 30 min at RT followed by dissociation into single cells. For P0, the back skin was incubated in 2.5 U/ml Dispase in EpiLife medium overnight. The epidermis was then manually separated from the dermis and incubated in Accutase for 30 min at RT followed by dissociation into single cells. For all time points, the dissociated cell suspension was strained with 40 µM filter and washed with media. Dead Cell Removal kit (Miltenyi Biotec) was used to remove dead cells prior to resuspension in 0.04% BSA (Thermo Fisher Scientific). Chromium Single Cell 3′ v1/v2 (10x Genomics) library preparation was then performed by the University of California, Irvine, Genomic High Throughput Facility (UCI-GHTF) according to manufacturer’s protocol. Immunofluorescence localization of markers Fresh frozen OCT 10 µM sections were incubated in acetone at −20 °C for 10 min, washed with TBS, fixed in 4% PFA for 10 min, and then washed with TBS three times. Tissues were then permeabilized using TBS with 0.3% TritonX-100 for 10 min and blocked in TBS with 0.5% BSA for 1 h. Primary antibodies, Krt14 (Abcam) and Krt10 (Covance), were diluted 1:1000 and incubated overnight at 4 °C. Secondary antibodies (Abcam, Life Technologies) were diluted 1:1000 and incubated at RT for 1 h. Images were acquired using a Keyence BZ-X700 fluorescent microscope. Fiji was used for image analysis. RNA fluorescent in situ hybridization (RNA-FISH) RNA-FISH was performed using the RNAscope Multiplex Fluorescent Detection Kit v1 according to manufacturer’s instructions on fresh frozen 10 µM thick OCT sections. All sections were counterstained with ProLong Gold antifade reagent with DAPI. Images were acquired on a Leica SP8 confocal microscope. To ensure that images were comparable, they were all processed the same maximum intensity projection and brightness. Three biological replicates were analyzed for each FISH staining experiment. Ex vivo Grhl3 −/− rescue experiment P0 WT and Grhl3 −/− littermate dorsal back skin (12 mm in diameter, n = 3 each) was harvested as described above. Each piece of skin was cut in half and each half was incubated ex vivo in 100 nM Wnt-C59 small molecule inhibitor (R&D Systems, 5148) or DMSO, in 3 ml of EpiLife medium (ThermoFisher Scientific, MEPICF500) without calcium for 48 h at 37 °C. We analyzed twenty images from each biological replicate of each condition using Fiji to measure the thickness of the epidermis. We determined the average thickness of each biological replicate and used one tailed paired student’s t -test to calculate the p -value. Sequencing Chromium Single Cell 3′ v1/v2 libraries were sequenced with either a Illumina HiSeq 2500 or a HiSeq4000 following the manufacturer’s protocol. Primary computational analysis Raw sequencing data were demultiplexed and processed using Cellranger (10× Genomics version 2.01) using MM10 reference provided by 10× Genomics. The number of cells, mean reads per cell and median number of genes per cell for each experiments are listed in Supplementary Data 1 . Cells were filtered and clustered using Seurat version 2.3.4 [19] . For E14.5 and E16.5, cells with <600 and >4800 genes detected were removed. For P0, cells with <900 and >7700 genes detected were removed. For all time points, genes that are expressed in <6 cells were removed, and cells with >10% mitochondrial genes detected were removed. Raw gene-cell matrices were normalized and scaled. Percentage of mitochondrial genes, and the number of unique molecular identifiers (UMI) were regressed out using the RegressOut function. High variable genes were identified using a x.low.cutoff of 0.0125 and y.cutoff of 0.5 on mean variance dispersion plot. Data for each developmental age were integrated with canonical correlation analysis (CCA) on each biological replicate followed by alignment of subspace of each sample. Louvain clustering was then performed on the integrated samples. Single-cell consensus clustering (SC3) was carried out using k = 2 for basal IFE subclustering. Cell cycle analysis was carried out in Seurat using a list of cell cycle genes from the Regev laboratory [20] . We performed integrative analysis of developing IFE cells across E14.5, E16.5, and P0 using Seurat V3 (version 3.0.1) according to its tutorial ( https://satijalab.org/seurat/v3.1/integration.html ). Briefly, we performed SCTransform normalization separately for each time point, selected 3000 informative features using SelectIntegrationFeatures and PrepSCTIntegration functions, and performed integration analysis for joint clustering. Cells were visualized using UMAP (Uniform Manifold Approximation and Projection) algorithm [36] . For the differential gene expression analysis of IFE cells across E14.5, E16.5, and P0, we employed the following three criteria to identify enriched genes for each developmental stage [37] : (i) the p -values from Wilcoxon rank-sum tests are less than 0.01, (ii) the log fold-changes are higher than 0.25, and (iii) the percentage of expressed cells in the tested developmental stage is higher than 25%. Gene Ontology enrichment analysis of the enriched genes was performed and visualized using ClusterProfiler R package [38] . The code for the integration analysis is provided in the Supplementary Software file . Pseudotemporal trajectory and RNA-velocity analysis Monocle version 2.10.1 was used to construct differentiation trajectories of IFE using the highly variable genes identified from Seurat package as an ordering filter. DDRTree was used for dimension reduction. No root state is specified and ordering was done in an unsupervised manner. The p -value cutoff for identifying pseudotime-dependent genes was p < 0.01. To model gene expression changes in pseudotime, we used scEpath package [14] , which first divides the pseudotime into ten equally spaced bins. Then the expression of each gene in each bin is estimated by the trimean of the expressions of this gene across all the cells located in this bin. Furthermore, scEpath smoothens the average expression of each gene using cubic regression splines. To study the temporal patterns and functional signatures of pseudotime-dependent genes, we performed k-medoids clustering based on the smoothed gene expression profiles, using Matlab function “kmedoids” with six clusters. We then created a heatmap to show the normalized-smoothed expression pattern of pseudotime-dependent genes. Genes within this heatmap were ordered such that nearest neighbors have similar expression profiles and genes within each cluster were ordered according to expression peak. The average expression pattern of each cluster is calculated by the trimean of smoothed expressions of all the genes in that cluster. For the pseudotemporal trajectory analysis of developing IFE across E14.5, E16.5, and P0, we projected cells into a low-dimensional space using a diffusion-based manifold learning approach PHATE [39] , with an input of the corrected data matrix from the integration analysis using Seurat V3. We then calculated the pseudotime of individual cells, identified the pseudotime-dependent genes and visualized pseudotemporal gene dynamics using scEpath package. 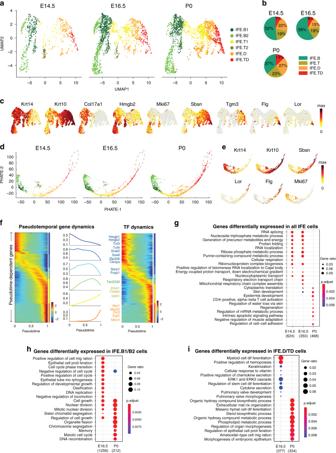Fig. 3: The IFE Differentiation program is already established at E14.5. aUMAP showing distribution of cell states as defined in the P0 IFE (Fig.1) in the developing IFE (E14.5, E16.5, and P0). We observe two transition populations, IFEE.T1 and IFE.T2, at E14.5 and E16.5. IFE.T2 cells are proliferating transition cells.bPie charts showing the proportion of major cell states at each developmental time point. IFE.B and IFE.TD decrease and increase, respectively, across development.cThe expression of the indicated differentiation and proliferation markers projected onto the combined UMAP for all three developmental time points ina.dPHATE maps of cell populations defined ina, showing pseudotime progression at each developmental stage. The gray circle emphasizes the extension of terminal differentiation at P0.eExpression of the indicated differentiation and proliferation markers onto the combined PHATE maps fromd.fLeft panel, expression heatmap and expression pattern of 2801 pseudotime-dependent genes from the combined PHATE maps fromd; these cluster into six gene modules. Right panel, expression heatmap of 149 pseudotime-dependent transcription factor (TF) genes from the combined PHATE maps fromc. Representative TFs from each gene modules are color-coded and indicated on the left. Gene lists in Supplementary Data1.gGene ontology categories of genes differentially expressed at each developmental stage in all IFE cells. Gene lists in Supplementary Data1.hGene ontology categories of genes differentially expressed at E16.5 and P0 in IFE.B1 and IFE.B2 cells. Gene lists in Supplementary Data1.iGene ontology categories of genes differentially expressed at E16.5 and P0 in IFE.D and IFE.TD cells. Gene lists in Supplementary Data1. Of note, the calculated pseudotime values were scaled ranging from 0 to 1. To discover key transcription factor programs responsible for cell states and state transitions during development, the transcription factors responsible for cell state transitions during epidermal differentiation were identified from the set of pseudotime-dependent genes based on the transcription factors annotated in AnimalTFDB [40] . 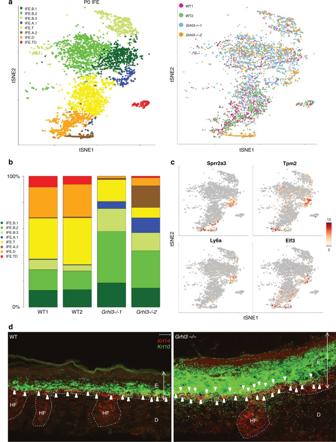Fig. 4: GRHL3 is required for suppressing aberrant basal IFE stem cells. atSNE plot showing WT andGrhl3−/−P0 IFE cells colored by clusters (left) and genotype (right).bBar plot showing the fraction of each IFE cell type in each sample. There is expansion of basal cells and reduction of differentiated/terminally differentiated cells inGrhl3−/−IFE.cGene expression levels of markers for the IFE.A1 population.Sprr2a3, Tpm2, Ly6a and Eif3are shown on a tSNE plot of the P0 IFE cells.dRepresentative RNA-FISH ofKrt14andKrt10transcripts in P0 WT andGrhl3−/−mouse epidermis; white arrows highlightKrt14/Krt10double-positive transition cells. Note the higher number of double-positive cells in theGrhl3−/−epidermis; also some transition cells are found in the spinous layer.N= 5. White broken line, basal lamina; E epidermis, D dermis, HF hair follicle. Scale bar = 10 µm. RNA-velocity analysis was performed using the velocyto pipeline ( https://github.com/velocyto-team/velocyto.R ) [21] . The “run10x” function was used on Cellranger ouputs to generate the loom files using default parameters, mm10 gtf file provided by 10× Genomics and repeat mask gtf file from the UCSC Genome Browser. For the RNA velocity estimation, we used the standard R implementation of velocyto and only considered cells that were part of the pseudotime. The cell-to-cell distance matrix was calculated based on the PCA embedding. RNA velocity was estimated using gene-relative model with k -nearest neighbor cell pooling ( k = 20). Embeddings from PCA and Monocle pseudotime analysis were used for velocity field projections. 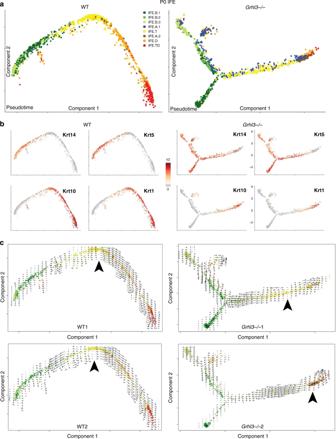Fig. 5: RNA velocity reveals a commitment point at the IFE.T/IFE.D transition. aPseudotime trajectories showing IFE differentiation going from IFE-B to IFE-T to IFE-D to IFE-TD for the two WT (left) and twoGrhl3−/−(right) P0 IFEs. TheGrhl3−/−differentiation trajectory has a branch which is attributed to the IFE-A1 population and expansion of basal, proliferating cells.bExpression ofKrt14,Krt5,Krt10, andKrt1projected on the pseudotime trajectory for the WT (left) and theGrhl3−/−(right) IFE.cRNA-Velocity analysis of the pseudotime trajectory of IFE cells for WT1, WT2,Grhl3−/−1,Grhl3−/−2. Direction of the arrows points to the fate the cells are heading toward; length of the arrows reflects how fast the cells are heading toward a particular fate. Note IFE differentiation is marked by a clear commitment point (arrowhead) and is a one-step, continuous process with no intermediary stages in the WT. In contrast, most cells fail to proceed through the commitment point (arrowhead) and transition cells show a propensity to go back to basal fate in theGrhl3−/−IFE. 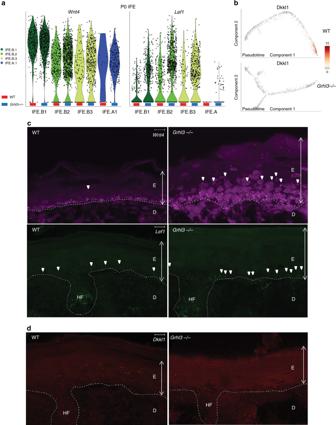Fig. 6: GRHL3 represses Wnt pathway gene expression in basal IFE cells. aViolin plot showing theWnt4(left) andLef1(right) expression for each cell among the basal cell types in the WT (both biological replicates) and theGrhl3−/−(both biological replicates) IFE. There is higher number ofWnt4-high andLef1-high cells in all basal and aberrant populations in theGrhl3−/−than in the WT.bExpression ofDkkl1projected on the pseudotime trajectory for the WT (top) and theGrhl3−/−(bottom) IFE. Note the decreased number of cells expressingDkkl1in theGrhl3−/−IFE.cRepresentative RNA-FISH images ofWnt4(upper panels) andLef1(lower panels) in WT andGrhl3−/−P0 epidermis. There is increasedWnt4expression and aberrant expression ofWnt4in cells above the basal layer inGrhl3−/−IFE as indicated with white arrowheads. There is increasedLef1expression in the basal layer in theGrhl3−/−IFE as indicated with white arrowheads.N= 3 WT andGrhl3−/−littermates. E epidermis, D dermis, HF hair follicle.dRepresentative RNA-FISH image ofDkkl1in WT andGrhl3−/−P0 epidermis. There is decreasedDkkl1expression in the suprabasal layers inGrhl3−/−IFE.N= 3 WT andGrhl3−/−littermates. White broken lines trace the basal lamina. E epidermis, D dermis, HF hair follicle. Scale bars = 10 µm. 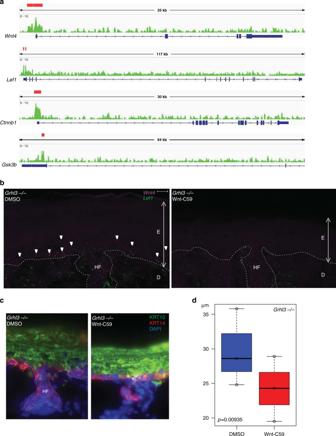Fig. 7: Wnt inhibition partially rescues epidermal hyperplasia in the Grhl3−/−IFE. aGRHL3 ChIP-seq signal on the indicated Wnt signaling genes in the E16.5 epidermis. The red bars represent significant peaks.bRepresentative RNA-FISH images ofWnt4(pink) andLef1(green) inGrhl3−/−P0 epidermis treated ex vivo with control (DMSO; left panel) or Wnt inhibitor (Wnt-C59; right panel). There is decreasedWnt4andLef1expression in the epidermis treated with the Wnt inhibitor. Arrowheads point to signal.N= 3 biologically independent samples each. White broken line traces basal lamina. E epidermis, D dermis, HF hair follicle.cRepresentative sections ofGrhl3−/−P0 epidermis treated ex vivo with control (DMSO; left panel) or Wnt inhibitor (Wnt-C59; right panel), representative image forN= 3 each. Krt14 staining, red; Krt10 staining, green; DAPI staining; blue; HF, hair follicle. There is decreased IFE thickening of the Wnt inhibitor treated epidermis. Scale bar = 10 µm.dSummary statistics for IFE thickness, mean and standard error for ex vivo Wnt inhibitor experiments.P-value was calculated with one-tailed studentt-test.N= 3 biologically independent samples each. Reporting summary Further information on research design is available in the Nature Research Reporting Summary linked to this article.